Atomically perfect torn graphene edges and their reversible reconstruction The atomic structure of graphene edges is critical in determining the electrical, magnetic and chemical properties of truncated graphene structures, notably nanoribbons. Unfortunately, graphene edges are typically far from ideal and suffer from atomic-scale defects, structural distortion and unintended chemical functionalization, leading to unpredictable properties. Here we report that graphene edges fabricated by electron beam-initiated mechanical rupture or tearing in high vacuum are clean and largely atomically perfect, oriented in either the armchair or zigzag direction. We demonstrate, via aberration-corrected transmission electron microscopy, reversible and extended pentagon–heptagon (5–7) reconstruction at zigzag edges, and explore experimentally and theoretically the dynamics of the transitions between configuration states. Good theoretical-experimental agreement is found for the flipping rates between 5–7 and 6–6 zigzag edge states. Our study demonstrates that simple ripping is remarkably effective in producing atomically clean, ideal terminations, thus providing a valuable tool for realizing atomically tailored graphene and facilitating meaningful experimental study. Manipulation of graphene edges at the atomic level is of fundamental importance in exploiting graphene’s recognized potential in next generation electronic, optical, mechanical and chemical devices [1] , [2] , [3] , [4] , [5] , [6] , [7] . For example, the electronic band-structure of graphene nanoribbons depends strongly not only on ribbon width but also on the detailed edge termination [1] , [2] , [3] , [4] . Zigzag (ZZ) and armchair (AC) graphene edges have distinct electronic states and scattering properties [1] , [2] , [3] , [4] , [5] , [6] as well as unique chemical properties [5] , [6] , [7] . Although theoretical studies [1] , [2] , [3] , [4] , [5] , [6] , [7] have shed light on important aspects of bare and functionalized graphene edges, experimental observations and manipulation of ‘ideal’ graphene edges at the atomic scale have been difficult to achieve, especially for suspended samples not influenced by substrate bonding and charging effects. Available investigations of graphene edges have revealed that edges are prone to intrinsic and extrinsic modifications such as atomic-scale defects, structural distortions, and inhomogeneous and often unintended chemical functionalization. For example, most top-down fabrication processes including lithography, oxidative unzipping and catalytic etching with metal result in highly defective edge structures [8] , [9] , [10] , [11] , [12] . Recently, anisotropic etching of graphene with hydrogen at elevated temperature has been used to produce nominally ZZ edges [13] , [14] but a direct atomic-scale characterization of the edge quality remains lacking. Bottom-up fabrication of graphene nanostructures has also yielded encouraging high-quality edge structure [15] , [16] but there are limitations in cleanly separating graphene from strongly interacting metal substrates. Obtaining an atomically precise and chirality-controlled graphene edge configuration is paramount to understanding truncated graphene’s intrinsic properties and in enabling many graphene applications. We have previously demonstrated that nicks in a tensioned suspended graphene membrane can be stimulated with an electron beam, thereby causing the membrane to catastrophically rupture or tear [17] . The direction of the tear (that is, crack) follows almost exclusively the AC or ZZ direction, at least when viewed at the micrometre scale (the AC direction is more prone to tearing than the ZZ direction) [17] . However, the edge quality or configuration at the atomic scale has hitherto not been determined. Indeed, the alignment of graphene edges with high symmetry directions (AC or ZZ) at the micrometre scale does not guarantee perfect edge structure at the atomic level [12] , [18] ; in principle, an edge that appears to be in the ZZ direction at the large scale could be composed of random (or collections of AC) edge structures at the atomic scale. Previous experimental edge studies of graphene include micro Raman spectroscopy [14] , [15] , [18] , scanning tunnelling microscopy [15] , [16] , [19] , [20] , [21] and transmission electron microscopy (TEM) [12] , [17] , [22] , [23] , [24] , [25] , [26] . Scanning tunnelling microscopy and TEM allow observations of graphene edges at the atomic scale including different electronic scattering properties and edge stability. Aberration-corrected TEM is an ideal tool for investigating graphene edges over relatively large areas with both atomic scale (sub-Å) spatial resolution and meaningful temporal resolution; it also eliminates unwanted substrate effects [12] , [17] , [22] , [23] , [24] , [25] , [26] . In this study, we employ aberration-corrected TEM to demonstrate that graphene edges created by in situ tearing of suspended monolayer graphene have clean, atomically smooth edges in the ZZ or AC directions with over 90% edge configuration fidelity. We also observe extended pentagon–heptagon (5–7) reconstruction at the ZZ edge and demonstrate reversible transformation of the entire edge between different reconstructions. The atomic edge configurations are monitored in real-time and the edge-configuration-dependent dynamics, and stability are analysed using both experiment and appropriate theoretical models. Effective activation barriers are extracted. 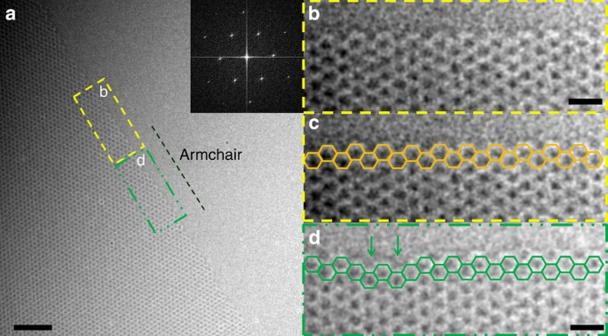Figure 1: Straight graphene torn edge with AC edge configuration. (a) Atomic resolution TEM image of a torn edge with AC configuration. The inset is the Fourier transform of the image. The yellow and green dashed boxes are the field of view for figure b and d, respectively. Scale bar, 2 nm. (b) The zoom-in image of the graphene edge showing a perfect AC edge. Scale bar, 0.5 nm. (c) The same TEM image with atomic structure overlay. (d) The zoom-in image of the graphene edge at a different location showing a segment with local irregularity. The arrows indicate the locations of four missing atoms. Scale bar, 0.5 nm. TEM imaging of torn graphene with AC and ZZ edges Figure 1 shows atomic resolution TEM images of a torn graphene edge nominally aligned with the AC lattice direction. The lower left side of Fig. 1a is a region of suspended single-layer graphene, whereas the upper right side of the image shows vacuum. The inset to Fig. 1a is the Fourier transform of the image from which the overall lattice orientation is determined. The main image in Fig. 1a was taken with an accumulated electron beam dose <10 7 e nm −2 so as to capture the pristine edge configuration, as produced by the in situ tearing process (see Methods for the detailed procedure). Notably, the torn graphene edge is extremely clean, regular and straight even at the atomic scale. Figure 1b shows a zoomed-in image near the edge, which reveals a perfect AC edge configuration (shown with atomic overlay in Fig. 1c ). Figure 1d shows another segment of the graphene edge where a slightly irregular edge shape is revealed, with carbon atom vacancy defects. In this (rare) segment, four carbon atoms are missing from the perfect edge configuration. Overall, the AC torn edge segments typically exhibit fractionally perfect edge structure over 90% (see Supplementary Table S1 for detailed data). We emphasize that in situ edge fabrication with electron beam stimulation in a clean (high vacuum) environment is key to obtaining atomically smooth edge structures without functionalization. Figure 1: Straight graphene torn edge with AC edge configuration. ( a ) Atomic resolution TEM image of a torn edge with AC configuration. The inset is the Fourier transform of the image. The yellow and green dashed boxes are the field of view for figure b and d, respectively. Scale bar, 2 nm. ( b ) The zoom-in image of the graphene edge showing a perfect AC edge. Scale bar, 0.5 nm. ( c ) The same TEM image with atomic structure overlay. ( d ) The zoom-in image of the graphene edge at a different location showing a segment with local irregularity. The arrows indicate the locations of four missing atoms. Scale bar, 0.5 nm. Full size image Extended ZZ torn edges with atomically smooth, ideal edge structure are also observed. 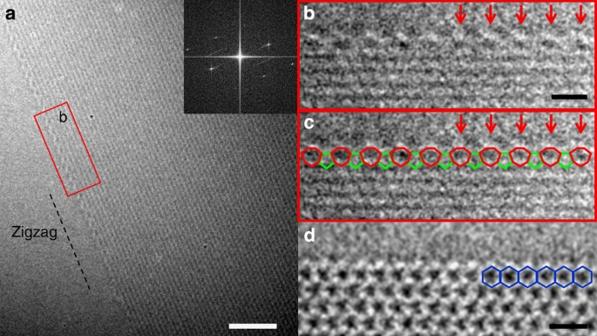Figure 2: Straight graphene torn edge with ZZ edge configuration. (a) Atomic resolution TEM image of a torn edge in ZZ direction. The inset is the Fourier transform of the image. The red box is the field of view for figure b. Scale bar, 2 nm. (b) Zoom-in image of the graphene edge. The red arrows indicate heptagon rings with 4.92 Å inter-ring distance. Scale bar, 0.5 nm. (c) The same figure with atomic overlay. The graphene edge shows a pentagon–heptagon (5–7) reconstructed ZZ edge configuration. (d) Graphene torn edge with pure (6–6) ZZ edge configuration (without reconstruction). The atomic edge configuration is overlaid at the right side of the image. Scale bar, 0.5 nm. Figure 2a shows an atomic resolution TEM image of a torn edge aligned in the ZZ lattice direction. Figure 2b is a zoomed-in image of the same graphene edge. Although in these images it is non-trivial to resolve the location of each carbon atom because of sample tilting and electron beam-induced mechanical instability, we observe that there is a clear periodic intensity pattern at the graphene edge with a periodicity of around 4.9 Å, as marked with red arrows in Fig. 2b . This intensity pattern originates from a previously predicted [5] , [6] pentagon–heptagon (5–7) reconstruction at the ZZ edge (shown with atomic overlay in Fig. 2c ). This reconstruction has been previously investigated via TEM over a limited range [22] , [24] , [27] . More clearly resolved atomic resolution images of 5–7 reconstruction are presented later in this manuscript (see Figs 3 and 4 ). The 5–7 reconstructed edge can be derived from the pure (6–6) ZZ edge with only local carbon bond rotations and has lower edge energy than the (6–6) ZZ edge [5] . The experimentally obtained image of a 6–6 ZZ edge (that is, without 5–7 reconstruction) is shown in Fig. 2d for comparison. The 6–6 ZZ edge shows an intensity pattern with the regular graphene lattice periodicity of 2.46 Å. Again, as demonstrated in Fig. 2 and Fig. 1 , tearing graphene is a highly effective method to obtain atomically clean, well-defined graphene edges of specified chirality. Figure 2: Straight graphene torn edge with ZZ edge configuration. ( a ) Atomic resolution TEM image of a torn edge in ZZ direction. The inset is the Fourier transform of the image. The red box is the field of view for figure b. Scale bar, 2 nm. ( b ) Zoom-in image of the graphene edge. The red arrows indicate heptagon rings with 4.92 Å inter-ring distance. Scale bar, 0.5 nm. ( c ) The same figure with atomic overlay. The graphene edge shows a pentagon–heptagon (5–7) reconstructed ZZ edge configuration. ( d ) Graphene torn edge with pure (6–6) ZZ edge configuration (without reconstruction). The atomic edge configuration is overlaid at the right side of the image. Scale bar, 0.5 nm. 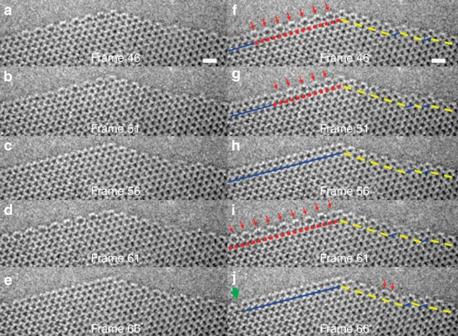Figure 3: A time series of TEM images of a graphene torn edge under electron beam. (a–e) A time series of TEM images of graphene edge. Each image is apart from each other by five frames. The left (right) segments have the ZZ (AC) edge configuration. Scale bar, 0.5 nm. (f–j) The same sequential TEM images with edge representations. The red arrow indicates a heptagon ring. The blue solid and red dotted lines represent 6–6 ZZ and 5–7 reconstructed ZZ edges, respectively. The yellow dashed lines show AC edge configuration. The green arrow injshows a vacancy defect. Full size image Figure 3: A time series of TEM images of a graphene torn edge under electron beam. ( a – e ) A time series of TEM images of graphene edge. Each image is apart from each other by five frames. The left (right) segments have the ZZ (AC) edge configuration. Scale bar, 0.5 nm. ( f – j ) The same sequential TEM images with edge representations. The red arrow indicates a heptagon ring. The blue solid and red dotted lines represent 6–6 ZZ and 5–7 reconstructed ZZ edges, respectively. The yellow dashed lines show AC edge configuration. The green arrow in j shows a vacancy defect. 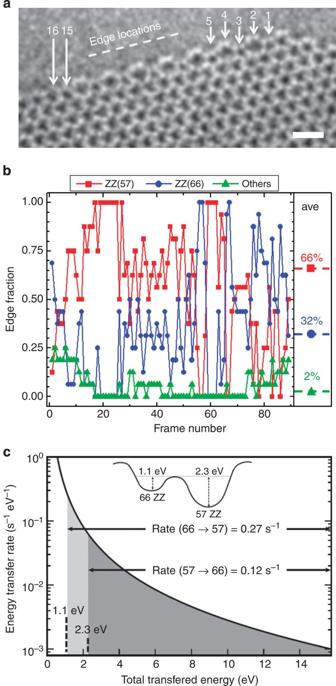Figure 4: Structural transitions between 6–6 and reconstructed 5–7 ZZ edge. (a) TEM image of graphene ZZ edge with assigned hexagon locations. The edge locations from 1 to 16 are monitored for structural transition frame by frame. Scale bar, 0.5 nm. (b) Time evolution of ZZ edge fraction during 89 time frames. The average occupied edge fraction (with frames from 20 to 70) is also shown. (c) Energy transfer rate to a single carbon atom as a function of transferred energy from electron beam. The total energy transfer rates shown by shaded areas give the effective activation barriers for flipping events between 5–7 and 6–6 ZZ edges. Inset shows the energy landscape of different ZZ edges. Full size image Figure 4: Structural transitions between 6–6 and reconstructed 5–7 ZZ edge. ( a ) TEM image of graphene ZZ edge with assigned hexagon locations. The edge locations from 1 to 16 are monitored for structural transition frame by frame. Scale bar, 0.5 nm. ( b ) Time evolution of ZZ edge fraction during 89 time frames. The average occupied edge fraction (with frames from 20 to 70) is also shown. ( c ) Energy transfer rate to a single carbon atom as a function of transferred energy from electron beam. The total energy transfer rates shown by shaded areas give the effective activation barriers for flipping events between 5–7 and 6–6 ZZ edges. Inset shows the energy landscape of different ZZ edges. Full size image Dynamics and stability of ZZ and AC edge configurations In situ fabricated atomically smooth ZZ and AC edge segments also provide excellent platforms for a detailed study of dynamics and stability of different edge configurations. Most previous TEM studies on graphene edges have relied on electron beam sputtering onto the graphene lattice to produce edge configurations (such as the edge around a growing hole) [22] , [24] , [28] . During sputtering, it is difficult to observe reversible transitions between bistable edge configuration states. In the present study extended edge configurations are readily available as pristine ZZ and AC edge configurations. We find that, under our electron illumination conditions, both AC and ZZ edges show dynamical effects, with the ZZ edge being much more active, as we now describe in detail. Figure 3 shows a time series of TEM images of a relatively rare torn graphene edge corner. This corner area is chosen for monitoring, as it shows flat ZZ and AC segments side by side, which facilitates a direct comparison of the dynamics. The electron beam exposure and read-out time are 0.5 and 1.3 s per frame, respectively. In Fig. 3a–e , five TEM images are shown where the sequential images are separated by five image frames. The upsloping left-side and down-sloping right-side segments within each panel show the ZZ and AC edge configurations, respectively. Overall, both graphene edges are quite stable to e-beam-induced sputtering at the experimental timescale (with beam current 2.1 (±0.1) × 10 6 e nm −2 s −1 ). Figure 3f–j shows the same sequential TEM images displayed with overlay edge representations. The red arrows indicate heptagon rings from 5–7 edge reconstructions. The observed periodicity of 4.92 Å in the ZZ region of Fig. 3f is in agreement with images shown in Fig. 2b,c , which confirms that the ZZ tear edge of Fig. 2 has 5–7 reconstruction. The red dotted and blue solid lines represent 5–7 reconstructed and 6–6 ZZ edges, respectively. As clearly shown in the time series of Fig. 3 , under the influence of the electron beam the ZZ edge frequently undergoes dramatic, extended and fully reversible structural transitions between a 5–7 reconstructed edge and a 6–6 ZZ edge. In particular, Fig. 3h,i shows that the left-side ZZ segment can have a 100% structure correlation with either 6–6 or 5–7 reconstruction. On the other hand, the AC edge (shown with yellow dashed lines) is relatively stable under the electron beam, consistent with previous theoretical calculations [29] . Edge dynamics at the AC edge are mainly related to embedded short ZZ edge segments (which result in a one-unit dynamic ‘step’ in the edge). To examine ZZ reconstruction dynamics in more detail, the left-side, upsloping extended ZZ segments shown in Fig. 3 are monitored for flipping between 6–6 and reconstructed 5–7 ZZ configurations, presented in Fig. 4 . We assign edge locations (from 1 to 16) in the ZZ segment as identified in Fig. 4a , and the edge configuration at each location is tabulated for a structural transition frame by frame (see Supplementary Movie 1 and Supplementary Table S2 for detailed data). Figure 4b shows the time evolution of the ZZ edge fraction during 89 time frames. The rapid and frequent transformations between 6–6 and reconstructed 5–7 edge structures are clearly shown in data. For example, the 6–6 ZZ edge transforms to a 100% reconstructed 5–7 edge in two frames (2.6 s) during the time frame 57–59. Green triangle data points in Fig. 4b represent other defect configurations such as adatom and vacancy defects. For the first 20 frames, part of the ZZ edge (edge locations 12~16) has an adatom (~0.2 in edge fraction) configuration and the edge starts to develop vacancy defects from frame 75 on. We find that the ZZ edge can effectively withstand knock-on damage for about ~50 time frames (65 s) in our experimental set-up. Overall, we observe more 5–7 reconstructed edge segments (66%) compared with 6–6 ZZ segments (32%) during frames 20–70. This is consistent with theoretical edge energy calculations, which show that the 5–7 reconstructed edge has the lower energy (~1.7 eV per a pair of hexagons) compared with the 6–6 ZZ edge [5] , [6] . Interestingly and importantly, the transformation to/from 5–7 ZZ configurations is a collective behaviour, with flips in one region highly correlated with nearby edge structure. We find that 5–7 reconstructions occur predominantly adjacent to pre-existing 5–7 locations. To quantify this behaviour, we first assign the 5–7 occupation value a ( x, t ) for a pair of carbon rings at the edge, with a ( x, t )=1 for a 5–7 ZZ edge pair and a ( x, t )=0 for a 6–6 ZZ pair. Here x (from 1 to 8) and t (from 20 to 70) represent different locations of carbon-ring-pair and time frames. We then define a probability function p for 5–7 reconstruction. This probability function calculates, for a given 5–7 reconstruction edge site, the probability that a nearest neighbour site (left and right locations) is occupied by 5–7 edges. If the 5–7 reconstruction occupies random sites along the ZZ edge, we expect that p is close to the average 5–7 edge fraction value, 66%. From our experimental data (see Supplementary Table S2 ), however, we obtain p =92%, which is significantly higher than the value with the random location assumption. This demonstrates a high degree of correlation between reconstructed 5–7 edge sites. Theoretical calculations have shown that the activation barrier for the first 5–7 edge reconstruction is ~0.8 eV and can be lowered with the presence of a 5–7 reconstruction nearby [30] . This lowered activation barrier by nearby 5–7 reconstruction is consistent with the observed correlation of 5–7 edge sites. We now consider the flipping rate at the ZZ edge between 6–6 carbon rings and 5–7 carbon rings, experimentally and theoretically. The activation barriers for the flipping are 0.8 eV (6–6=>5–7) and 2.4 eV (5–7=>6–6) [5] , [30] , which are significantly higher than the thermal energy. Therefore, in our experiment, the high-energy incident electron beam (80 keV) provides the energy for the transitions between 6–6 and 5–7 rings. The experimentally obtained flipping rates are 0.26 s −1 (6–6=>5–7) and 0.12 s −1 (5–7=>6–6), with a ratio R (6–6=>5–7)/(5–7=>6–6)~2.3. Using the cross-section for Coulomb scattering between an incident electron and a carbon atom [31] , [32] , we can estimate the total cross-section of scattering events where the energy above the threshold energy (0.8 eV or 2.4 eV) is transferred to a carbon atom (see the Supplementary Note 1 for the detailed calculations). Under our experimental condition ( j =2 × 10 6 e nm −2 s −1 ), we obtain rates of 0.38 s −1 (6–6=>5–7) and 0.11 s −1 (5–7=>6–6), which gives a rate ratio R =3.5 in good agreement with the experimental flipping rate ratio. (We assume that all the scattering events with energy transfers above the threshold energy result in a carbon ring flip process.) We find that thermal lattice vibrations [33] do not significantly change the atomic displacement rate and expected flipping rates. After taking the lattice vibrations into account, we obtain flipping rates of 0.44 s −1 (6–6=>5–7) and 0.13 s −1 (5–7=>6–6), with a ratio R ~3.4 (please see Supplementary Note 2 for detailed calculations). Using the experimentally observed flipping rates, we can also estimate the effective activation barriers for 6–6=>5–7 and 5–7=>6–6 transformations. Figure 4c shows the energy transfer rate to a single carbon atom as a function of transferred energy from the electron beam of 80 keV. We find certain effective cutoff energies, which reproduce experimentally obtained flipping rates (areas under the curve from the cutoff energy to maximum transfer energy). Using this procedure, we estimate that the effective activation energy barrier for the 6–6=>5–7 flip is 1.1 eV, whereas for the 5–7=>6–6 flip it is 2.3 eV (corresponding energy transfer rates are shown by shaded areas in Fig. 4c ). When we take thermal lattice vibrations into consideration [33] , the effective activation energy barriers increase by~0.2 eV (1.3 eV for 6–6=>5–7 and 2.5 eV for 5–7=>6–6). These effective activation energies are close to the calculated energy barriers required for these transformations (0.8 eV and 2.4 eV) [5] , [30] . One should note that here we have only considered the beam-induced displacement effect as the energy transfer mechanism and omitted other mechanisms. In fact, investigations of energy transfer mechanisms in electron microscopy are now actively pursued. They include ultrafast electron microscopy with ps of time resolution to address non-equilibrium phonon excitations and subsequent long wavelength atomic motion in thermalization processes [34] , the role ionization processes [35] and heating effects [36] . The inclusion of other mechanisms in our analysis can result in larger values for the estimated activation energies (see Supplementary Note 3 for discussion on other types of possible energy transfer mechanisms). In conclusion, we demonstrate that torn graphene edges produced by e-beam-induced rupture along ZZ or AC directions are exceptionally clean and straight even at the atomic scale. The ZZ edge can be completely and reversibly flipped between two different metastable configurations, one with pure hexagons at the edge, the other with previously predicted 5–7 reconstructions. Flipping rates and activation energies are consistent with theoretical modelling. With the observed high-energy barriers, we believe that the pure AC edge, and both of the ZZ-based edges, can be locked in and remain stable at room temperature. Materials Graphene is obtained by chemical vapour deposition (CVD) on polycrystalline copper (99.8% Alfa Aesar, Ward Hill, MA) with a growth temperature 1035 °C (ref. 37 ). After synthesis, graphene is transferred to Quantifoil holey carbon TEM grids by a clean transfer process [17] . We use Na 2 S 2 O 8 solution to etch the copper substrate. The CVD graphene sample is mostly monolayer with the average grain size of above 5 μm (ref. 38 ). The CVD graphene is suitable for preparing suspended graphene samples with large quantity, which enables us to systematically study in situ tearing of graphene edges. Atomic resolution TEM The atomic resolution TEM images of graphene edge were obtained with the TEAM 0.5 at the National Center for Electron Microscopy, Lawrence Berkeley National Laboratory. The microscope is equipped with image Cs aberration corrector and monochromator and was operated at 80 kV. The TEM image was taken at the over-focus 10 nm, which allows an optimal imaging condition with the bright atom contrast. In situ tearing of graphene and image acquisition were performed with vacuum pressures below 5 × 10 −8 Torr near the sample. For single-shot TEM images ( Figs 1 and 2 ), we went through the following steps to minimize the electron beam-induced damages to graphene torn edges. As shown in Supplementary Fig. S1 , we identify a pre-existing tear on suspended graphene at low magnifications. Once we find an area of interest, we temporarily block the electron beam. With a higher magnification, we set a focus and proper imaging setting on a sample area far away from the identified tear region. Then we move to a region where we expect to find an in situ -fabricated torn edge as shown in Supplementary Fig. S1a . The extended tear is usually prone to mechanical instability such as vibration, which prevents atomic resolution imaging of torn edge. The graphene tear around an edge of carbon support generally has better mechanical stability and allows atomic resolution imaging. How to cite this article: Kim, K. et al. Atomically perfect torn graphene edges and their reversible reconstruction. Nat. Commun. 4:2723 doi: 10.1038/ncomms3723 (2013).